Deformation-induced structural transition in body-centred cubic molybdenum Molybdenum is a refractory metal that is stable in a body-centred cubic structure at all temperatures before melting. Plastic deformation via structural transitions has never been reported for pure molybdenum, while transformation coupled with plasticity is well known for many alloys and ceramics. Here we demonstrate a structural transformation accompanied by shear deformation from an original <001>-oriented body-centred cubic structure to a <110>-oriented face-centred cubic lattice, captured at crack tips during the straining of molybdenum inside a transmission electron microscope at room temperature. The face-centred cubic domains then revert into <111>-oriented body-centred cubic domains, equivalent to a lattice rotation of 54.7°, and ~15.4% tensile strain is reached. The face-centred cubic structure appears to be a well-defined metastable state, as evidenced by scanning transmission electron microscopy and nanodiffraction, the Nishiyama–Wassermann and Kurdjumov–Sachs relationships between the face-centred cubic and body-centred cubic structures and molecular dynamics simulations. Our findings reveal a deformation mechanism for elemental metals under high-stress deformation conditions. When a material is loaded under stress, the accumulating elastic energy eventually sets off dissipative processes, such as plastic deformation. These processes are generally mediated by dislocation slip and deformation twinning or stress-assisted phase transformations. It is the nature of materials to take an easy deformation route; however, sometimes the high-cost paths must be taken when the easy deformation path is suppressed or bypassed. Among these deformation mechanisms, stress-assisted phase transformation is often an efficient outlet to accommodate the imposed straining, such as in transformation-induced plasticity steels [1] , [2] and shape memory alloys [3] . Phase transformations under straining have mostly been observed in materials with polymorphs [4] , [5] , [6] , [7] , [8] (such as iron with α-Fe, γ-Fe and ε-Fe). However, there are also materials, such as elemental molybdenum (Mo) with a body-centred cubic (bcc) structure, for which no other polymorphs have been observed. Indeed, computer calculations have predicted that alternative crystalline lattices of Mo, for example, a face-centred cubic (fcc) phase [9] , [10] , would have an energy much higher (0.2–0.4 eV per atom) [11] than that of bcc Mo. Thus, a fundamental question regarding these materials is whether their deformation can ever be coupled with a structural transformation that leads to the emergence of new (metastable) crystalline lattices/forms. In the present work, we report the direct observation of two sequential structural transformations in Mo in response to enhanced external loading. Here, refractory Mo is a powerful example that demonstrates that even for a highly stable bcc crystal, when the material (or a local region) is subjected to very high shear stresses and other plastic deformation routes (such as twinning) are suppressed or bypassed, the crystalline structure can be forced to change to release the local stress concentration. Specifically, the energetically uphill bcc-to-fcc transition becomes viable in Mo when driven by sufficiently high applied stresses. Bcc-fcc-bcc phase transformation under tensile loading In situ tensile tests were conducted on a pure multi-grain Mo film inside a transmission electron microscope (TEM) at room temperature (for details, see the Methods section and Supplementary Fig. 1 ). High stresses (and stress gradients) are expected in the region ahead of a crack tip (in our sample configuration, {010} is the crack plane and <001> is the direction of the crack front), providing the driving force for deformation and structural change. Time-resolved high-resolution TEM (HRTEM) images were recorded on digital videotape at 10 frames per second ( Supplementary Movie 1 ). Some frames were extracted, as shown in Fig. 1a–d . The loading direction of the tensile stress is denoted by a black arrow in Fig. 1a , and the area is located just ahead of a crack tip (on the left outside the HRTEM images in Fig. 1 ). The HRTEM image at t =0 s ( Fig. 1a ) and the corresponding fast Fourier transformation (FFT) pattern ( Fig. 1e ) reveal the <001> orientation of the bcc Mo. With the application of tensile stress, part of the <001> crystal transforms into a new grain with <111> orientation (see the corresponding FFT patterns in Fig. 1f,g ). With increasing loading, the newly formed grain grows rapidly ( Fig. 1b–d and Supplementary Movie 1 ). Note that the new <111>-oriented grain (hereafter, called bcc2; Fig. 1h ) abruptly occurs inside the original <001>-oriented matrix (hereafter, called bcc1), which is equivalent to a grain rotation of as large as 54.7°. 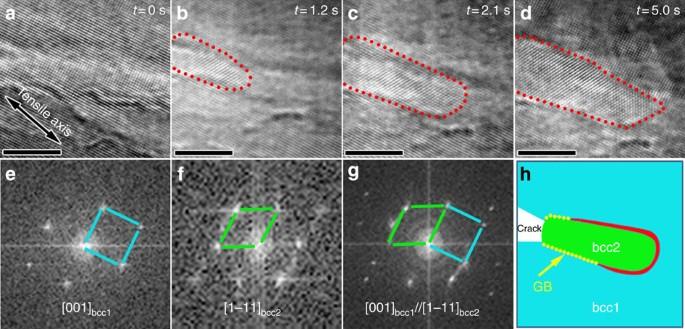Figure 1:In situelectron microscopy observations under tensile loading. (a–d) Time-resolved high-resolution transmission electron microscopy (HRTEM) images taken along the <001> direction of bcc Mo recorded att=0, 1.2, 2.1 and 5.0 s, respectively. A <111>-oriented grain formed and grown inside the <100>-oriented matrix is outlined by red dots. Scale bar, 5 nm. (e–g) FFT patterns of HRTEM images from the matrix (bcc1), the newly formed grain (bcc2) and both the matrix and newly formed grain, respectively. (h) A schematic illustration showing the distribution of bcc1 and bcc2 crystals. Figure 1: In situ electron microscopy observations under tensile loading. ( a – d ) Time-resolved high-resolution transmission electron microscopy (HRTEM) images taken along the <001> direction of bcc Mo recorded at t =0, 1.2, 2.1 and 5.0 s, respectively. A <111>-oriented grain formed and grown inside the <100>-oriented matrix is outlined by red dots. Scale bar, 5 nm. ( e – g ) FFT patterns of HRTEM images from the matrix (bcc1), the newly formed grain (bcc2) and both the matrix and newly formed grain, respectively. ( h ) A schematic illustration showing the distribution of bcc1 and bcc2 crystals. Full size image High-angle annular dark-field scanning TEM (HAADF-STEM) imaging was used for structural characterization. This technique, which uses incoherent electrons, allows direct imaging of atomic locations that is free of contrast reversals over a large range of sample thickness or objective lens defocus, thereby overcoming the uncertainties caused by dynamical diffraction, delocalization and interference in HRTEM imaging [12] . In addition, atomic-resolution STEM images are sensitive to crystal orientation [13] , [14] , such that the lattice would appear amorphous even when the sample orientation deviates by only ~1° from a zone axis. Nanodiffraction, with the electron beam diameter focused to ~1 nm, provides an additional probe to identify the structure in local regions of interest. The HAADF-STEM image in Fig. 2a reveals three regions (I, II and III) that exhibit distinctly different features in the lattice images. This general sample area is one bcc Mo grain imaged along its <001> zone axis. It is therefore surprising to observe three regions that do not appear to have the same structure or orientation. This observation is the first hint that suggests that some structural changes may have occurred during deformation. The angle- β between two basic vectors ( x and y ) is measured for all the intersecting atomic planes across the entire image of Fig. 2a , and the β -distribution obtained is plotted in Fig. 2b . Unexpectedly, three peaks emerge at ~88.9°, 70.3° and 60.6° for regions I, II and III, respectively, while only the first peak at β =~90° (for region I) is expected for the bcc Mo imaged in the <001> direction. In fact, each region is predominantly characterized by a specific β . The value of β =~60° for region III can be matched with bcc Mo if the viewing direction coincides with the <111> orientation. Most notably, region II has a characteristic angle- β very close to 70.5°, which is unusual for the bcc lattice but is consistent with an fcc lattice viewed in the <110> direction. 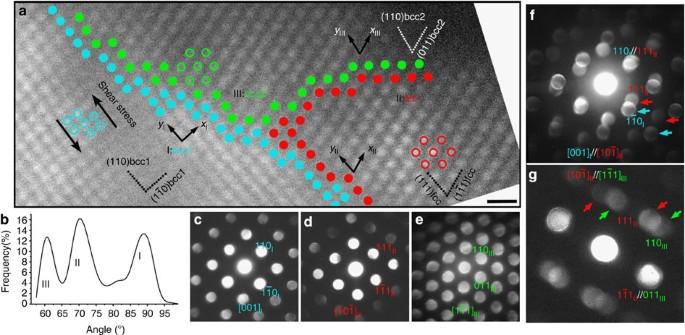Figure 2: Three structural variations in Mo. (a) Atomic-resolution high-angle annular dark-field scanning transmission electron microscopy (HAADF-STEM) image showing regions I, II and III with different crystal structures or orientations. Atoms adjacent to the boundaries between the regions are represented using different colours: blue for the original <001>-bcc1 region, red for the <110>-fcc region and green for the <111>-bcc2 region. Scale bar, 0.5 nm. (b) Distribution of the measured angle-βbetween two basic vectors (xandy) in the entire imaged area. (c–g) The electron NDPs from regions I, II, III, I+II and II+III, respectively. The blue, red and green arrows indicate diffraction discs from region I, II and III, respectively, infandg. Figure 2a can therefore be taken as the first indication that a different structure has emerged in region II, and that the structure is fcc-like. The original image of Fig. 2a without marks is also presented in Supplementary Fig. 2 to show the three regions and interfaces between them. A similar HAADF-STEM image proving the existence of the fcc-like structure at another crack tip is presented in Supplementary Fig. 3 , and a corresponding discussion is provided in Supplementary Note 1 . Figure 2: Three structural variations in Mo. ( a ) Atomic-resolution high-angle annular dark-field scanning transmission electron microscopy (HAADF-STEM) image showing regions I, II and III with different crystal structures or orientations. Atoms adjacent to the boundaries between the regions are represented using different colours: blue for the original <001>-bcc1 region, red for the <110>-fcc region and green for the <111>-bcc2 region. Scale bar, 0.5 nm. ( b ) Distribution of the measured angle- β between two basic vectors ( x and y ) in the entire imaged area. ( c – g ) The electron NDPs from regions I, II, III, I+II and II+III, respectively. The blue, red and green arrows indicate diffraction discs from region I, II and III, respectively, in f and g . Full size image To more convincingly identify the structural changes across the three regions, electron nanodiffraction patterns (NDPs) were acquired from each region (I, II and III) and bi-region (I+II and II+III) in Fig. 2a , as shown in Fig. 2c–g , respectively. Figure 2c–e , which were acquired from three individual regions, exhibit three distinctly different zone-axis diffraction patterns, providing clear evidence that three well-defined structures/orientations are present. Figure 2c indicates that region I consists of a bcc matrix with a lattice parameter a =0.312 nm along the [001] axis (bcc1), and Fig. 2e reveals that region III is again bcc; however, the pattern appears to be taken along the [1-11] zone axis, confirming the presence of a new bcc orientation (bcc2), rotated by 54.7° from region I. Region II, notably, generates diffraction spots in Fig. 2d , which are consistent with the [10-1] pattern of an fcc structure with lattice parameter a =0.409 nm. The indexing of these NDPs is explained in detail in Supplementary Note 2 , which explains that the NDPs can explicitly distinguish an fcc Mo from bcc Mo crystals. After tilting the fcc phase ~19° away from the original [10-1] direction, another fcc NDP that is [10-2] oriented is obtained ( Supplementary Fig. 6 ), which agrees well with the angle of 18.4° between the [10-1] and [10-2] axes of a fcc crystal. Nevertheless, owing to the geometry of the fcc phase at the crack tip, after tilting ~19° away from the initial orientation, the small volume fcc crystal unavoidably overlapped with the relatively large bcc grain at the crack tip along the direction of the incident electron beam. Therefore, the NDP was acquired from the overlapped fcc ([10-2]-oriented) and bcc1 ([114] and [113]-oriented) lattices in this direction. The indexing detail of this NDP is described in Supplementary Note 3 . These diffraction results are consistent with the indications from the β -angle distributions discussed above: there are three separate structures/orientations in the deformation zone, bcc1, fcc and bcc2. The presence of an fcc region II is the most noteworthy. Figure 2f,g are NDPs of the bi-regions I+II and II+III, respectively, taken across the interface of two regions. Each NDP from the bi-region reveals only the simple superposition of two individual diffraction patterns. The orientation relationship between bcc1, fcc and bcc2 can be readily derived from the NDPs. For bcc1 and fcc, Fig. 2f (and Fig. 2a ) suggests (110) bcc1 //(111) fcc and [001] bcc1 //[10-1] fcc , which correspond to the Nishiyama–Wassermann (N–W) [15] orientation relationship in a bcc←fcc transition. Meanwhile, the orientation relationship between fcc and bcc2 is revealed by Fig. 2g : (1-11) fcc //(011) bcc2 and [10-1] fcc //[1-11] bcc2 , which correspond to the Kurdjumov–Sachs (K–S) [16] relationship between bcc and fcc. A similar scenario where two different sets of orientations of a bcc crystal are connected with/through one fcc orientation, although for a different material, was enumerated by He et al . [17] The match with the well-established bcc←fcc crystallographic relationship reinforces the structural identification above: it is reasonable for region II to be in an fcc structure as an intermediate state bridging the two bcc orientations. We can therefore view the three regions as arising from the following sequence of structural transformation driven by enhanced shear stress: the <001>-oriented bcc1 crystal first transitions into the fcc state and subsequently transforms into the new <111>-oriented bcc2 structure, which finally undergoes ~15.4% elongation along the shear direction. The same stress-induced phase-transition sequence was predicted by molecular dynamics (MD) simulations for nanocrystalline α-iron [18] . Note that the relationship between bcc1 and bcc2 is [001] bcc1 //[1-11] bcc2 with an ~10° difference between the (110) bcc2 and (110) bcc1 planes, with bcc2 being equivalent to a lattice rotation of 54.7° relative to the original bcc1 lattice. We now discuss the evidence that indicates that the new fcc structure is a metastable phase. First, this phase has a ubiquitous presence: the same particular characteristics as those in Fig. 2 and Supplementary Fig. 3 are often detected by STEM images and NDPs at different {010}<001> crack tips. Ahead of bcc2 crystals, a ‘region II’ exists with the most-probable angle of 70.8°±1.2° by statistical analysis (see details in Supplementary Note 2 and Supplementary Table 2 ), and a well-defined set of nanodiffraction spots consistent with the fcc structure is observed. Second, NDPs from two different zone axes of the crystal are obtained, which can sufficiently define the fcc structure. Third, the phase has appreciable dimensions: the fcc patches are as wide as 13 atomic layers in Fig. 2a and have an ~4 × 8 nm 2 area in Supplementary Fig. 3 . Fourth, our observations also rule out the possibility that the phase is merely because of continuous elastic distortion of the original bcc1 lattice. It has been reported that continuous distortion should induce a series of continuously varying unit cell parameters [19] . If the new structural region II was a distorted bcc structure continuously from region I to III, the angle- β of each region II would be equally distributed between 60° and 90° rather than the observed most-probable value of ~70.5°. Therefore, all the TEM results suggest that the new fcc structure is a metastable state into which the bcc phase is driven. Further support for a deformation-driven transformation (bcc1→fcc→bcc2) is provided by MD simulations, which were performed on single crystalline bcc Mo with the same initial crack configuration {010}<001> as that in the experiment (for the simulation details, see the Methods section). 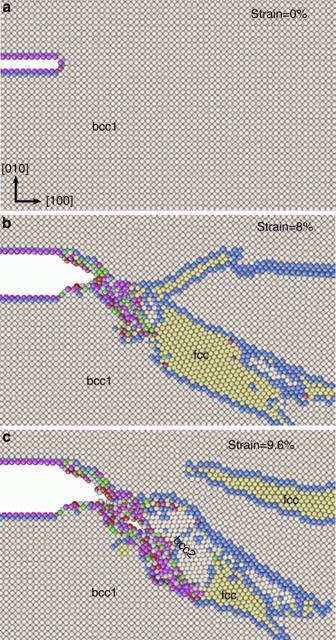Figure 3: Snapshots showing the structural transition during the molecular dynamics (MD) simulation. (a) The simulation configuration with a crack. (b) Two fcc regions develop inside the bcc1 matrix. (c) The lower fcc patch converts into bcc2. The atoms are coloured according to their coordination number, white: 14 (bcc), blue: 13, yellow: 12 (fcc), maroon: 11, green: 10 and pink: 9. See the Methods section for explanations. Figure 3a–c present a succession of snapshots acquired during the simulation. As the tensile strain increases, two patches of fcc Mo emerge (for more details, see the phase identification and analysis descriptions in the Methods section). The atomistic details provided by the MD approach allowed us to observe how the structural transitions proceed: the fcc phase originates from bcc1 via successive atomic shear along <110> and small shuffles ( Fig. 3b ; for details, see Supplementary Note 4 and Supplementary Figs 7a–d and 8 ). The resultant orientations follow the N–W relationship, which is consistent with the earlier experimental results (also see Fig. 2f ). In Fig. 3c , a new bcc region (bcc2) nucleates with an orientation that is different from that of bcc1. The bcc2 region grows with increasing loading at the expense of fcc via atomic shear along the {111} fcc plane ( Fig. 3c ; for details, see Supplementary Note 4 and Supplementary Fig. 7e–h ), resulting in the K–S relationship between bcc2 and fcc (comparable with Fig. 2g ). Details regarding the atomic shear mechanism of the bcc1→fcc→bcc2 phase transitions are schematically illustrated in Supplementary Fig. 9 and described in Supplementary Note 4 . The mechanisms of the bcc1→fcc and fcc→bcc2 phase transformations are the N–W and K–S phase transformation mechanisms, respectively. This series of deformation behaviour, with phase transitions involved and the resultant rotation of the lattice orientation from bcc1 to bcc2, corroborates our experimental observations. The mechanisms revealed lend important support to the phase evolution routes observed in real-world samples. In particular, we note that the MD analysis helps to ascertain that the new structure is indeed a distinct metastable phase with fcc crystal symmetry. Figure 3: Snapshots showing the structural transition during the molecular dynamics (MD) simulation. ( a ) The simulation configuration with a crack. ( b ) Two fcc regions develop inside the bcc1 matrix. ( c ) The lower fcc patch converts into bcc2. The atoms are coloured according to their coordination number, white: 14 (bcc), blue: 13, yellow: 12 (fcc), maroon: 11, green: 10 and pink: 9. See the Methods section for explanations. Full size image Fcc-to-bcc phase transformation under unloading Upon unloading the imposed stresses, the higher energy fcc structure is prone to transitions toward the low-energy bcc state, as expected. In some cases, the fcc structure transforms back to bcc1. In the meantime, portions of the bcc2 region can re-orient to join the bcc1 matrix (to reduce the interfacial energy). One example case is illustrated in Fig. 4a ( t =0 s) and Fig. 4b ( t =228 s), showing HRTEM images during unloading. The blue, red and green dots represent the original bcc1 phase, the intermediate fcc phase and the bcc2 phase, respectively. At t =0 s, a clear and large area of fcc structure in thin-plate shape mainly on the {110} bcc plane is observed in Fig. 4a , which is in accordance with the elasticity theory. Comparing Fig. 4a,b 228 s later, almost the entire fcc lath and a portion of the bcc2 lattice have transformed back to the original orientation of bcc1. To confirm that these imaged regions indeed have the structures claimed here, three images were selected from different regions (black-boxed areas 1, 2 and 3) in Fig. 4a and enlarged in Fig. 4f–h . To help understand these experimentally acquired images, they were compared with simulated images of bcc Mo along the [001] and [111] zone axes ( Fig. 4i,k ), and fcc Mo along the [110] zone axis ( Fig. 4j ). The experimentally acquired and simulated images match exceptionally well, indicating that the black-boxed areas 1, 2 and 3 are indeed bcc1 along <001>, fcc along <110> and bcc2 along <111>, respectively. 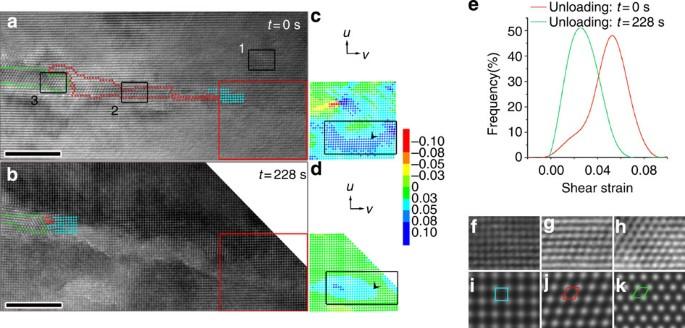Figure 4: Time-resolved HRTEM images showing structural changes during unloading. (a,b) HRTEM images att=0 s (a) andt=228 s (b). The blue, red and green dots represent the original bcc1, the fcc and bcc2 structure, respectively. Scale bar, 5 nm. (c,d) The lattice shear distortion determined from the red-boxed areas in the left HRTEM images analysed by the lattice distortion analysis (LADIA) software. (e) Quantitative shear strain analysis of the black-boxed regions incandd, respectively. The frequency is the proportion of lattice points with a certain shear strain within the total number of lattice points in the black-boxed areas. (f–h) Enlarged images of the black-boxed areas 1, 2, and 3 ina, respectively. (i,k) Simulated HRTEM images of bcc Mo along the [001] and [111] zone axes, respectively, with a lattice parameter ofa=0.3147, nm. (j) Simulated HRTEM image of fcc Mo along the [110] zone axis with a lattice parameter ofa=0.4030, nm (ref.41). The simulations were conducted for an acceleration voltage of 300 kV, a spherical aberration coefficient of 1.2 mm and a focus value of −33 nm. Figure 4 is thus further evidence supporting the presence of three structural zones as illustrated using HAADF-STEM in Fig. 2a . In this case, the relationships between bcc1 and bcc2 are [001] bcc1 //[1-11] bcc2 and (110) bcc1 //(110) bcc2 ( Fig. 4a,f–k )), which are variants of the relationship in Fig. 2a , in which [001] bcc1 //[1-11] bcc2 and an angle of ~10° is observed between the (110) bcc2 and (110) bcc1 planes. The occurrence of two bcc2 variants (both revealed convincingly by HAADF-STEM images, for example, Fig. 2a and Supplementary Fig. 10a ) is because of the two equivalent (111) and (1-11) planes in the [10-1] zone axis of the fcc phase serving equally as shear transformation planes, again supporting the fcc symmetry of region II. The atomic formation process of the two bcc2 variants is explained in Supplementary Note 4 and Supplementary Fig. 9 . Figure 4: Time-resolved HRTEM images showing structural changes during unloading. ( a , b ) HRTEM images at t =0 s ( a ) and t =228 s ( b ). The blue, red and green dots represent the original bcc1, the fcc and bcc2 structure, respectively. Scale bar, 5 nm. ( c , d ) The lattice shear distortion determined from the red-boxed areas in the left HRTEM images analysed by the lattice distortion analysis (LADIA) software. ( e ) Quantitative shear strain analysis of the black-boxed regions in c and d , respectively. The frequency is the proportion of lattice points with a certain shear strain within the total number of lattice points in the black-boxed areas. ( f – h ) Enlarged images of the black-boxed areas 1, 2, and 3 in a , respectively. ( i , k ) Simulated HRTEM images of bcc Mo along the [001] and [111] zone axes, respectively, with a lattice parameter of a =0.3147, nm. ( j ) Simulated HRTEM image of fcc Mo along the [110] zone axis with a lattice parameter of a =0.4030, nm (ref. 41 ). The simulations were conducted for an acceleration voltage of 300 kV, a spherical aberration coefficient of 1.2 mm and a focus value of −33 nm. Full size image Stress state analysis The next question concerns the stress states of the bcc Mo crystal when the deformation-induced structural changes occur. To demonstrate that the sample region of interest indeed experiences enhanced stress concentration, quantitative strain analysis was performed using the lattice distortion analysis (LADIA) package [20] , [21] on time-resolved HRTEM images. An angle- θ is used to describe the lattice shear strain in the bcc1 crystal at the crack tip (see details in the Methods section). The angle- θ is defined as the included angle between two basic vectors u (1/2[110]) and v (1/2[1-10]) in the (001) plane ( Fig. 5 ). 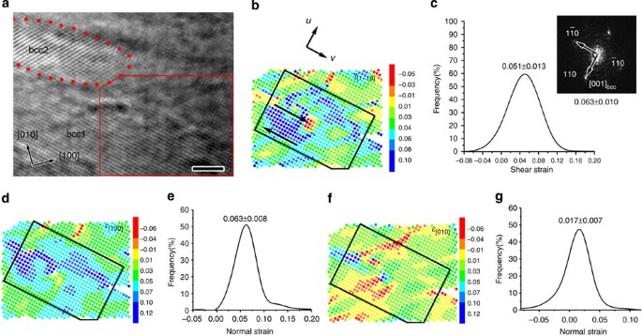Figure 5: Strain analysis from lattice distortions in HRTEM image. (a) An HRTEM image att=1.5 s extracted from the same movie asFig. 1a–d. Scale bar, 2 nm. (b) Lattice shear distortion along [1-10] determined from the red-boxed bcc1 area ina, analysed using the LADIA program. (c) Quantitative distribution of shear strain for atoms in the black-boxed region inb. The inset incis the FFT of the HRTEM image corresponding to the black-boxed area inb. (d,f), Lattice normal distortion along [100] and [010], respectively, determined from the red-boxed bcc1 area ina. The atoms are coloured according to strain scale: colours for positive values represent tensile strain, and colours for negative values represent compressive strain. (e,g) Quantitative distribution of tensile strain along [100] and [010], respectively, for atoms in the black-boxed region inb. The frequency is the fraction of lattice points with a certain strain out of the total number of lattice points in the black-boxed area. The error bars represent the s.d. Figure 5a was extracted from Supplementary Movie 1 ( t =1.5 s). The lattice distortion of the red-boxed area in Fig. 5a is shown in Fig. 5b . The shear strains shown in Fig. 5b using different colours suggest that the local Mo matrix is under a shear stress (indicated by black arrows) that originated from the external tensile stress. Figure 5c displays the quantitative lattice distortion profile for the black-boxed region (used as a lattice strain gage) in Fig. 5b , indicating that the mean value of shear strain is 0.051±0.013 (all the error bars here represent the s.d.). The resolution here represents an estimated value for the static observations that correspond to individual HRTEM images [22] , [23] . Alternatively, using a FFT (the inset in Fig. 5c ) from the HRTEM image area corresponding to the black-boxed region in Fig. 5b , the average angle between the (110) and (1-10) planes was measured [24] to be 93.6±0.6°, corresponding to a shear strain of 0.063±0.010. This shear strain is consistent with, within the margin of error, that given by the LADIA analysis. Therefore, the local elastic shear stress is ~8 GPa, based on the shear modulus of 126 GPa [25] . Furthermore, the local normal strains in the viewing plane were also analysed. The normal strain distributions of the red-boxed area in Fig. 5a along [100] and [010] are shown in Fig. 5d,f , respectively, in which the atoms are coloured according to the strain scale: colours for positive values represent tensile strain and those for negative values represent compressive strain. These figures reveal that the local normal stresses along the two directions in front of the crack tip are all tensile stresses. The corresponding quantitative strain profiles presented in Fig. 5e,g indicate that the mean elastic tensile strains are 0.063±0.008 and 0.017±0.007, respectively. Accordingly, the tensile stresses along [100] and [010] are estimated to be ~20.7±2.6 GPa and ~5.6±2.3 GPa, respectively, given that the Young’s modulus is 329 GPa (ref. 25 ). These normal stresses would correspond to a shear stress of ~7.6 GPa, roughly estimated using the equation (G [010] -G [100] )/2, which is consistent with the measured shear stress along [1-10] of ~8 GPa. Owing to the projection view of the HRTEM image, the normal stress perpendicular to the viewing plane is not available by LADIA analysis. Thus, an MD simulation was used for the analysis of the three-dimensional normal stresses. The strain results for the [001], [100] and [010] directions are presented in Fig. 6b–d , respectively. 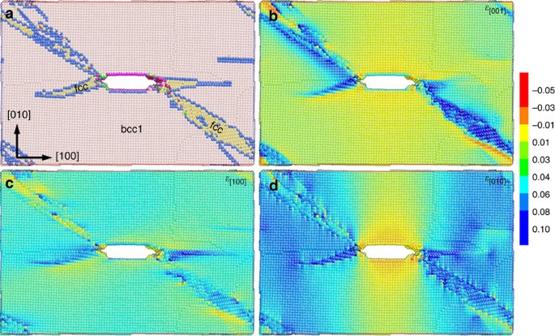Figure 6: Strain analysis by MD simulation. (a) A snapshot showing the bcc1 and fcc phases during tensile loading. The atoms are coloured according to their coordination number, white: 14 (bcc), blue: 13, yellow: 12 (fcc), maroon: 11, green: 10 and pink: 9. (b–d) The normal strain mapping along [001], [100] and [010], respectively. The atoms are coloured according to the strain scale: colours for positive values represent tensile strain, and colours for negative values represent compressive strain. The scale bar is shown in the right colour column. Figure 6a shows the structural features in different regions at the same moment with the three strain maps during the MD simulation. In Fig. 6a , the atoms are coloured according to their coordination number (white: 14 (bcc), blue: 13, yellow: 12 (fcc), maroon: 11, green: 10 and pink: 9). In Fig. 6b–d , the atoms are coloured according to the strain scale: colours for positive values represent tensile strain and colours for negative values represent compressive strain. It is apparent that tensile stresses are also present along the [100] and [010] directions in front of the crack tip, which agrees with the LADIA analysis results. For the [001] direction, no significant tensile stress is observed. Therefore, such a three-dimensional stress state in front of the crack tips is more complicated than the hydrostatic stress and uniaxial stress states, which likely explains the occurrence of the bcc1→fcc phase transition. Figure 5: Strain analysis from lattice distortions in HRTEM image. ( a ) An HRTEM image at t =1.5 s extracted from the same movie as Fig. 1a–d . Scale bar, 2 nm. ( b ) Lattice shear distortion along [1-10] determined from the red-boxed bcc1 area in a , analysed using the LADIA program. ( c ) Quantitative distribution of shear strain for atoms in the black-boxed region in b . The inset in c is the FFT of the HRTEM image corresponding to the black-boxed area in b . ( d , f ), Lattice normal distortion along [100] and [010], respectively, determined from the red-boxed bcc1 area in a . The atoms are coloured according to strain scale: colours for positive values represent tensile strain, and colours for negative values represent compressive strain. ( e , g ) Quantitative distribution of tensile strain along [100] and [010], respectively, for atoms in the black-boxed region in b . The frequency is the fraction of lattice points with a certain strain out of the total number of lattice points in the black-boxed area. The error bars represent the s.d. Full size image Figure 6: Strain analysis by MD simulation. ( a ) A snapshot showing the bcc1 and fcc phases during tensile loading. The atoms are coloured according to their coordination number, white: 14 (bcc), blue: 13, yellow: 12 (fcc), maroon: 11, green: 10 and pink: 9. ( b – d ) The normal strain mapping along [001], [100] and [010], respectively. The atoms are coloured according to the strain scale: colours for positive values represent tensile strain, and colours for negative values represent compressive strain. The scale bar is shown in the right colour column. Full size image A similar LADIA analysis has been applied to the unloading procedure, as shown in Fig. 4c–e . At the moment of unloading, the residual lattice shear distortion remains large in the vicinity of the newly formed fcc grain ( Fig. 4c ). After the fcc region and a part of the bcc2 region transformed back to bcc1, the lattice shear distortion decreases significantly, as illustrated by comparing the areas indicated by the black arrow in Fig. 4c,d . Quantitative lattice distortion profiles ( Fig. 4e ) from the black-boxed areas in Fig. 4c,d indicate that the mean values of shear strain are 0.054±0.005 and 0.028±0.009, respectively, before and after the reversed transformation. Because fcc Mo is of higher energy than bcc Mo [11] , it is expected that a relatively small fluctuation would be sufficient to cause the fcc-to-bcc transition. The phase transformation coupled with shear deformation in Mo has never before been observed, even though many studies regarding the deformation behaviour of Mo have been reported, for example, Mo nanofiber-tensile [26] or nanopillar-compression [27] , [28] experiments. What special conditions must exist for the bcc→fcc phase transition in Mo to be observed in this work? First, an extremely high applied shear stress >7 GPa in this work) is necessary to thermodynamically drive the low-energy-state bcc Mo into the high-energy-state fcc Mo, which is different from the stress state used in the high pressure research community [29] , [30] . In conventional uniaxial compression and tensile experiments, it is normally difficult to apply an extremely high stress on bulk Mo samples because the active dislocation slipping and twinning release the stress easily. However, in certain nanometer-scaled samples [26] , [27] , [28] as well as at the front of the crack tips in the in situ tensile TEM experiment, an extremely high stress, ~20 GPa in some cases, has been applied (at least in some stress concentration regions) when few dislocation activities and no twinning activities were involved. Second, driven by the large elastic strain energy (a few kJ per mol), the bcc→fcc phase transformation coupled with shear plastic deformation may occur in these Mo samples. The bcc→fcc phase transformation process will progress rapidly to the final bcc state (such as bcc2 in this work) without any confinements for holding the high-energy-state fcc Mo. In this case, the intermediate fcc phase is difficult to detect. Considering the large lattice orientation change (a grain rotation of ~54.7° in this work) and massive shear deformation strain (a tensile strain of ~15.4% in this work) achieved at the moment of the bcc→fcc→bcc phase transitions, catastrophic yielding (elongation or collapse) may be observed during the uniaxial tensile or compression processes if the phase transitions occurred. Catastrophic yielding at very high stress has been observed in Mo nanofiber-tensile [26] and Mo nanopillar-compression [27] , [28] experiments. Note that most of the collapses for the bcc Mo exhibited an asymmetrical shear shape, which is not formed by twinning [27] and is difficult to explain using a dislocation self-multiplication mechanism [31] . At the crack tips, the deformation area is localized and well confined; therefore, the intermediate fcc phase may be strained to be sustainable for being observed and characterized, as shown in this work. Third, twinning deformation, another important massive shear deformation mechanism, has been suppressed/bypassed in this work. For our {010}<001> crack, none of the {112} twinning planes are parallel to the crack front <001>, such that twinning on the {112} plane is suppressed. The atomic-resolution STEM image and NDPs in Fig. 2a also confirm that the bcc1 and bcc2 regions here do not have a twinning relationship (see details in the Methods section). For comparison, when changing the crack orientations from {010}<001> to {001}<110> (see Methods section), the MD simulations ( Supplementary Fig. 11 ) and experiments ( Supplementary Fig. 12 ) indicate that the high-cost bcc→fcc structural transformation was absent, and twinning processes were activated at the crack tips under the loading condition, which is consistent with a previous calculation [32] . In summary, the collective evidence from the HAADF-STEM imaging, NDPs, N–W and K–S crystallographic relationships, two variant crystallographic relationships between bcc1 and bcc2, and MD simulations lead us to conclude that a deformation pathway in Mo is available through structural transformations via a transitional metastable fcc state. The two-step phase transition, bcc1→fcc→bcc2, constitutes a new route for lattice rotation during deformation. The eventual bcc2 corresponds to a rotation of the lattice orientation by as large as 54.7°, and an ~15.4% tensile strain is achieved with respect to the original bcc1 crystal in the absence of conventional mechanisms for lattice reorientation, such as deformation twinning, grain boundary sliding and grain rotation, and movements of dislocations and disinclinations. Considering that nanometer-sized materials/devices are likely to experience some extremely complicated stress conditions in their applications, a phase transformation coupled with large shear deformation or catastrophic yielding may occur in high-stress deformation conditions, even for some elemental metals without polymorphs (such as Mo in this work). Thus, this mechanism may be important for nanomaterials deformed under high-stress conditions. Sample preparation and TEM and STEM characterization Polycrystalline Mo (99.9 wt.% pure) acquired from Alfa Aesar (Ward Hill, MA, USA) was used for the experiments. In situ TEM tensile specimens were thinned by ion milling and then glued onto the centres of Mo substrates with dimensions of 9 mm × 2.5 mm × 60 μm ( Supplementary Fig. 1 ). TEM, STEM and electron nanodiffraction investigations were conducted on an FEI Tecnai F30 and Titan 80–300 with an STEM resolution of ~0.136 nm. In situ tensile tests were performed at room temperature using a Gatan model 654 single-tilt straining holder. The tensile loading was controlled by applying intermittent displacement. Time-resolved HRTEM images of the deformed area were recorded on digital video at 10 frames per second; hence, the time resolution of the experiment was 0.1 s. Details about MD simulations and the fcc phase identification MD simulations were used to investigate the atomic processes of the phase transitions and grain rotation in bcc Mo. The embedded-atom-method interatomic potential [33] used in the present simulation has been broadly used in previous investigations for Mo [34] , [35] , [36] , [37] , [38] and has proven to be one of the most appropriate potentials to simulate the mechanical behaviour of Mo [34] , [35] , [36] , in particular plastic deformation near crack tips [37] , [38] . The simulation box contained 1.5 million atoms, with dimensions of 62.9 nm × 9.4 nm × 37.8 nm along the [100], [010] and [001] directions, respectively. A slab of 930 atoms was removed from the centre of the box, followed by subsequent relaxation, to produce an initial microcrack with a crack tip configuration of {010}<001> ({010} is the crack plane and <001> is the crack front). Tensile deformation was then imposed along the [010] direction at a constant strain rate of 10 7 s −1 at 300 K. Periodic boundary conditions were imposed in all three directions. The temperature and pressure were controlled using the Nose–Hoover thermostat [39] and Parrinello–Rahman method [40] , respectively. The time step was 1 fs. Simulations were repeated in smaller boxes with 1, 0.8 and 0.4 million atoms under strain rates ranging from 10 6 to 10 9 s −1 , and similar phase transition processes were observed. According to the atomic coordination number and local symmetry, atoms in bcc and fcc lattices can be identified. Furthermore, the fcc lattice regions were examined manually from their characteristic crystallographic orientations and close-packed plane. Atoms without bcc or fcc symmetry were also observed and were mostly located at boundaries. All the atoms are coloured according to their coordination numbers, that is, white: 14 (in bcc lattice), blue: 13, yellow: 12 (in fcc lattice), maroon: 11, green: 10 and pink: 9. For comparison, a different crack tip configuration of {001}<110> ({001} is the crack plane and <110> is the crack front) was set as the initial configuration for the MD simulation. Unlike the occurrence of the phase transitions bcc1→fcc→bcc2 for the {010}<001> crack tip configuration given above, a twinning process occurs at the crack tip configuration of {001}<110>, as observed in Supplementary Fig. 11 . The {112}<111> twins are observed in the MD simulations under this crack configuration, which agrees with the calculation in previous works [32] and our experimental results ( Supplementary Fig. 12 ). For the {001}<110> crack configuration, there are two {112} twining planes parallel to the crack front, and the twinning shear occurred easily to form the deformation twins. Therefore, the phase transitions bcc1→fcc→bcc2, a high-cost deformation path, will not be preferred in this case. It is well known that the strain rate in MD simulation is much higher than in real experiments. Thus, are the MD simulation results credible? First, note that when plastic deformation in metals is highly localized, the strain and the strain rate are both significantly increased in the local regions compared with the average value imposed on the sample. MD simulations indeed focus on these regions. Second, MD simulations are usually used to study non-diffusive processes, such as in the present paper, for which the simulation results on plastic deformation are far less sensitive against strain rate compared with experiments where various thermal-activated events occur. For instance, the present MD simulation results were obtained under strain rates ranging from 10 6 to 10 9 per second. The orientation relationships between bcc1 and bcc2 The <111> axis of the bcc2 crystal is parallel to the <001> axis of the bcc1 crystal. This relationship cannot be formed by {112}<111> twining. For a bcc structure, {112}<111> is a common twinning system in which {112} is the twin plane and <111> is the twinning direction. Being content with this twin relationship, the <001> direction in the matrix is parallel to the <221> direction of the twin lattice, that is, <221> twin //<001> matrix . However, in our observed results, all the newly formed bcc2 crystals have the relationship <111> bcc2 //<001> bcc1 to the bcc1 matrix. In particular, the atomic-resolution STEM images (for example, Fig. 2a ) reveal that [001] bcc1 is precisely parallel to [1-11] bcc2 , which is ~16° away from the [2-21] bcc2 zone axis and further away from other <221> bcc2 . Considering that atomic-resolution STEM images are very sensitive to the crystal orientation with an accuracy of ~1° (ref. 14 ), the possibility of a twin relationship of <221> bcc2 //<001> bcc1 was ruled out. Therefore, the bcc2 grains with [001] bcc1 //[1-11] bcc2 cannot be attributed to twinning products. The ultra-high lattice rotation under the crack configuration of {010}<001> in the present paper does not correspond to the twinning process. In other tensile experiments with different crack configurations, we observed the twinning process during deformation. Supplementary Figure 12 presents an HRTEM image taken under the {001}<110> crack configuration along the [110] bcc direction, showing two bcc crystals with the {112}<111> twinning relationship. This finding is consistent with the MD simulation result ( Supplementary Fig. 11 ), but is completely different from the lattice rotation discussed in the present paper. Two bcc2 variants of an fcc symmetry phase As described in the Results section, two orientation relationships exist between the matrix bcc1 and the newly formed bcc2 grains: [001] bcc1 //[1-11] bcc2 and (110) bcc1 //(110) bcc2 , as observed in Figs 1 and 4a , and [001] bcc1 //[1-11] bcc2 and (110) bcc2 deviating from (110) bcc1 about ~10°, as observed in Fig. 2a . Some bcc2 grains remained nearby the crack after the tensile sample broke. Supplementary Fig. 10 presents HAADF-STEM and HRTEM images of the bcc2 grains taken along the [1-11] bcc2 direction, in which the two bcc2 variants with the two different orientation relationships to the bcc1 matrix are observed, respectively. After excluding the possibility of {112}<111> twinning, the two bcc1-bcc2 orientation relationships indicated that two bcc2 variants resulted from the fcc-to-bcc phase transition. Based on the experimental observations ( Fig. 2a,f ), the structural transition from bcc1 to fcc corresponds to the N–W orientation relationship with [001] bcc1 //[10-1] fcc and (110) bcc1 //(111) fcc , which is driven by the applied stress. The transition from the high energy fcc phase back to the bcc phase corresponds to the K–S relationship with [10-1] fcc //[1-11] bcc2 and (1-11) fcc //(011) bcc2 ( Fig. 2a,g ). In this case, the (011) bcc2 plane is parallel to the (1-11) fcc plane; thus, a small angle of ~10° exists between (110) bcc2 and (110) bcc1 while [001] bcc1 //[1-11] bcc2 ( Fig. 2a and Supplementary Fig. 10c ). Considering the crystallographic symmetry of the fcc and bcc structures and the driving force of the fcc-to-bcc transition, the (111) fcc plane is equivalent to the (1-11) fcc plane for the fcc→bcc phase transition. Thus, there is an equivalent chance for the (110) bcc2 plane to be parallel to the (111) fcc plane, for which the other variant with the K–S relationship of [10-1] fcc //[1-11] bcc2 and (111) fcc //(110) bcc2 is obtained, as observed in Fig. 4a . Consequently, bcc2 grains with the orientation relationships of [001] bcc1 //[1-11] bcc2 and (110) bcc1 //(110) bcc2 are observed in the sample ( Supplementary Fig. 10a,b ). Owing to the equivalent {111} planes in the fcc structure, two bcc2 variants result from the fcc-to-bcc phase transition. Conversely, the two bcc2 variants verified the plane equivalence in the new phase, which provides further evidence for the existence of the fcc phase during deformation. Strain analysis by LADIA The LADIA package was used to analyse the stress states of the bcc Mo crystal during the loading and unloading of tensile stress. We use the angle ( θ ) between the basic vectors u (1/2[110]) and v (1/2[1-10]) in the (001) plane to describe the lattice shear strain of the bcc1 crystal ( Figs 4c,d and 5b ). The undistorted angle- θ 0 between u and v is 90° for bcc1. However, under a shear stress, the angle- θ will vary with the lattice distortion. For instance, θ becomes an acute angle when a shear stress, such as that shown in Fig. 5b (by two parallel arrows), is applied or becomes an obtuse angle when sheared in the opposite direction. Thus, the strain state of a bcc crystal during loading and unloading can be determined by the LADIA analysis. The quantitative LADIA results for the black-boxed areas in Figs 4c,d and 5b are presented in Figs 4e and 5c , respectively. Here, the frequency is the proportion of lattice points with a certain shear strain within the total number of lattice points in the black-boxed areas. How to cite this article: Wang, S. J. et al . Deformation-induced structural transition in body-centred cubic molybdenum. Nat. Commun. 5:3433 doi: 10.1038/ncomms4433 (2014).